Displays of paternal mouse pup retrieval following communicative interaction with maternal mates Compared with the knowledge of maternal care, much less is known about the factors required for paternal parental care. Here we report that new sires of laboratory mice, though not spontaneously parental, can be induced to show maternal-like parental care (pup retrieval) using signals from dams separated from their pups. During this interaction, the maternal mates emit 38-kHz ultrasonic vocalizations to their male partners, which are equivalent to vocalizations that occur following pheromone stimulation. Without these signals or in the absence of maternal mates, the sires do not retrieve their pups within 5 min. These results show that, in mice, the maternal parent communicates to the paternal parent to encourage pup care. This new paradigm may be useful in the analysis of the parental brain during paternal care induced by interactive communication. Parenting is an energetically costly activity in mammals, and mothers and fathers have a different impact on their offspring’s parental care [1] . Outstanding questions are what factors determine male parental care, and how such care can be encouraged [1] , [2] , [3] , [4] . At the neuroscientific level, this question may be addressed by studying the molecular and neuronal function of the male parental brain [2] , [4] , [5] , [6] . The vertebrate parental brain has been studied in species that typically provide biparental care [7] ; these include prairie voles [5] , [6] , California mice [8] , [9] and marmosets [10] , [11] . These species exhibit social recognition, female/male bonding and pup retrieval, and these behaviours correlate with various hormone levels, including oxytocin, vasopressin, prolactin, oestrogen and cortisol [4] , [5] , [6] , [7] , [8] , [9] , [10] , [11] , [12] , [13] , [14] , [15] , [16] , [17] . In contrast, laboratory mice, rats and hamsters are not monogamous, and males are not spontaneously parental [4] , [5] , [8] , [12] , [15] , [17] . However, if male and female mice are forced to live together for long periods in a small cage, the male will inevitably be found in the nest with the offspring providing protection and warmth. This process is similar to a process referred to as ‘senitization’, which has been described in male rats [17] . Many vertebrates use species-specific means to communicate information [16] , [18] , [19] , [20] , [21] , [22] , [23] . In the mouse, one important communication and recognition signal is ultrasonic (>20 kHz) vocalization (USV [20] , [22] ). Other important means of communication in this species include visual and olfactory input, body contact, and pheromones in urine and tears [19] . USVs emitted by adult mice have been considered a component of both the male sexual behavioural repertoire and social recognition in female–female interactions [22] , [23] , [24] , [25] , [26] . Female mice rarely emit USVs to males, but USVs emitted by pups increase pup survival because they are perceived as a signal to initiate maternal parental care [20] , [22] , [24] , [25] , [26] . Therefore, it is of interest to test whether adult females emit USVs during stressful conditions, such as dam–sire–pup separation, as a quantitative message to parental males or pups. Here, we address the following questions about parental behaviour in non-biparental males of mice: first, we wanted to determine how parenting is induced or altered by the environment. Second, we wanted to determine whether mice can be motivated to be parental. In the present work, we determine the precise conditions associated with paternal parental behaviour in ICR outbred mice. We found that the maternal parent communicates vocally to the paternal parent to encourage pup care, revealing new insights into interactive communication in rodents. Maternal behaviour in home cages The basic experimental paradigm used in this study for assessing parental care is shown in Fig. 1 . Virgin male and female ICR mice were paired and continuously housed together in a standard mouse maternity cage ( Fig. 1a ). The cages were left undisturbed during the first 3–5 days after the birth of the first litter produced by each pair; during this time, the new dam mainly nursed the pups. The new sire cared for the pups in the nest in the absence of the dam or together with her. Care from the sire involved mainly licking behaviour and huddling over or near the pups; the time devoted to maternal behaviour during the 30 min before the separation tests described below is shown in Fig. 2a . During this pre-separation period, which represents a well-adapted situation, paternal retrieval behaviours (returning pups to the nest by carrying them in the mouth and burrowing under wood chips, as part of nest building) were very infrequent. As specific motor behaviours were induced upon reunion of the parents and pups after removal or relocation in parent–pup separation, we used retrieval as the main criterion [7] , [17] for maternal behaviour by new and experimentally naïve sires (one trial per male) unless otherwise stated. 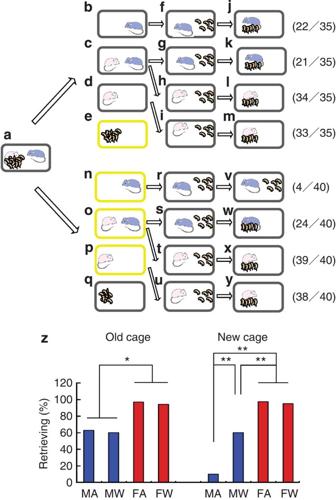Figure 1: The parental care test in ICR mice. Schematic representations of the parental care test in a mated pair isolated in an old (b–d) or new (n–p) cage. After cohabiting with their pups as a family unit (a), the parents were separated from the pups for 10 min (b–e) and then reunited with five pups (f–i). Subsequent pup retrieval behaviour was then observed (j–m), and the number of family members (new sire or dam) showing retrieval was scored and expressed as a percentage in (z) (one trial per mouse). In (a–m), the pups were placed in a new holding box (e, yellow), and the parents remained in the old box (b–d, grey) during the separation period (n=35 families each). The number on the right indicates the sires or dams with retrieval out of subjects tested. In (a,n–y), the pups remained in the old cage (q, grey), while the parents (separately or together) were placed in new isolation boxes (n–p, yellow;n=40 families each). The number on the right indicates sires or dams with retrieval out of subjects tested. (z) Percentages of males (M) and females (F) showing retrieval behaviour upon reuniting after separation alone (MA or FA) or with the mate (MW or FW). Left, results of the experiments in sires, dams, and sires and dams that were separated for 10 min in old cages. Right, results of the experiments on animals separated into new cages. Fisher’s test, two-tailed, *, **P<0.01, 0.001, respectively). Figure 1: The parental care test in ICR mice. Schematic representations of the parental care test in a mated pair isolated in an old ( b – d ) or new ( n – p ) cage. After cohabiting with their pups as a family unit ( a ), the parents were separated from the pups for 10 min ( b – e ) and then reunited with five pups ( f – i ). Subsequent pup retrieval behaviour was then observed ( j – m ), and the number of family members (new sire or dam) showing retrieval was scored and expressed as a percentage in ( z ) (one trial per mouse). In ( a – m ), the pups were placed in a new holding box ( e , yellow), and the parents remained in the old box ( b – d , grey) during the separation period ( n =35 families each). The number on the right indicates the sires or dams with retrieval out of subjects tested. In ( a , n – y ), the pups remained in the old cage ( q , grey), while the parents (separately or together) were placed in new isolation boxes ( n – p , yellow; n =40 families each). The number on the right indicates sires or dams with retrieval out of subjects tested. ( z ) Percentages of males (M) and females (F) showing retrieval behaviour upon reuniting after separation alone (MA or FA) or with the mate (MW or FW). Left, results of the experiments in sires, dams, and sires and dams that were separated for 10 min in old cages. Right, results of the experiments on animals separated into new cages. Fisher’s test, two-tailed, *, ** P <0.01, 0.001, respectively). 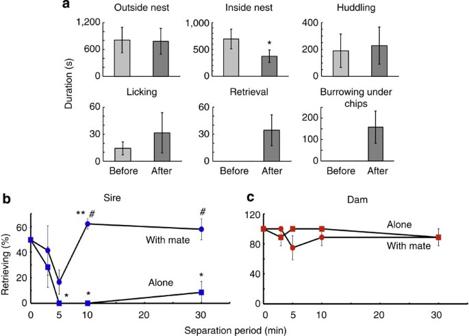Figure 2: Parental behaviour and the temporal nature of retrieval behaviour. (a) Duration of various maternal behaviours performed by the sires in their home cages for 30 min before and after 10-min separation from pups in a new cage together with their mates. Mean±s.e.m. (n=5 sires; Student’st-test, *P<0.05). (b,c) Effects of cohabitation duration on retrieval behaviour in parental males (b) and females (c). Parents were isolated alone (squares) or together with their mates (circles) in a new cage for 3, 5, 10 or 30 min. Subsequently, the animals showing retrieval upon reunion in the old cages were counted. In two different separation groups, 24 families were examined at each time point. Experiments were grouped for statistical analysis, and one-way ANOVA followed by Bonferroni’spost hoctest was performed (F4,15=3.56, *P<0.05 from 0 min, **P<0.01 from 5-min cohabitation). Student’st-test for two different separation groups at 10 and 30 min,#P<0.01. Full size image Figure 2: Parental behaviour and the temporal nature of retrieval behaviour. ( a ) Duration of various maternal behaviours performed by the sires in their home cages for 30 min before and after 10-min separation from pups in a new cage together with their mates. Mean±s.e.m. ( n =5 sires; Student’s t -test, * P <0.05). ( b , c ) Effects of cohabitation duration on retrieval behaviour in parental males ( b ) and females ( c ). Parents were isolated alone (squares) or together with their mates (circles) in a new cage for 3, 5, 10 or 30 min. Subsequently, the animals showing retrieval upon reunion in the old cages were counted. In two different separation groups, 24 families were examined at each time point. Experiments were grouped for statistical analysis, and one-way ANOVA followed by Bonferroni’s post hoc test was performed ( F 4,15 =3.56, * P <0.05 from 0 min, ** P <0.01 from 5-min cohabitation). Student’s t -test for two different separation groups at 10 and 30 min, # P <0.01. Full size image Parental behaviour after parent–pup separation To test male and female parental behaviour after parent–pup separation, the pups of each litter were removed and placed in a separate holding cage for 10 min ( Fig. 1e ) while one or both of the parents were left in the original cages ( Fig. 1b–d , respectively). Five pups from the litter were then returned to the nursing cage but placed in a remote area away from the nest. In nearly all of the trials, when dams were re-united with their pups, they rapidly gathered the pups and resumed nursing: 34 dams isolated with mates retrieved out of 35 families tested (97.1%, Fig. 1c ) or 33 dams isolated alone out of 35 families (94.3%, Fig. 1d ) in old cages for 10 min. Surprisingly, in more than half the trials, the sire assumed a similar parental role irrespective of whether he had remained in the home cage on his own (22 sires retrieved out of 35 families tested or 62.9%; Fig. 1b ) or had been removed with the dam (21 sires out of 35 subjects or 60%; Fig. 1c ). Retrievals by the sires and dams were significantly different (Fisher’s test, two-tailed P <0.01; Fig. 1z , left). These results demonstrate that male retrieval behaviour in the home cage is mate-independent, probably because pup and/or dam cues remained. Paternal care after separation into new clean cages The retrieval behaviour shown by males in Fig. 1j might have been induced by the nursing cage environment during the parent–pup separation. To assess this possibility, the paradigm used to obtain the data in Fig. 1a–m was reversed; the pups were left in the home cage ( Fig. 1q ) while the parents were placed in a clean cage for 10 min, either singly or together ( Fig. 1n–p ). Under these conditions, female parental care was unchanged. Thirty-eight dams isolated alone retrieved out of 40 families tested (95.0%; Fig. 1p ) versus 39 dams isolated with mates out of 40 subjects (97.5%; Fig. 1o ). Male parental care was also undiminished when the sires were housed with the females. Twenty-four sires retrieved out of 40 families tested (60.0%; Fig. 1o ); however, it was significantly reduced when the sires were housed separately from the dams. Four sires retrieved out of 40 families tested (10.0%; Fig. 1n ); Fisher’s test, two-tailed ( P <0.001; Fig. 1z right). Other sires’ parental behaviours, such as the duration spent outside or inside the nest, huddling and licking, and burrowing under chips, during the 30 min preceding the 10-min separation with their mates in new cages and after reunion in the old cages were examined ( Fig. 2a ). The duration spent outside the nest, huddling and licking, was unchanged, while duration of time spent inside the nest was significantly decreased because the sires initiated vigorous retrieving and burrowing behaviours upon reunion. As a control, the sires’ behaviour for 30 min before and after separation of sire alone was observed. These sires showed a similar locomotive pattern of behaviour ( Supplementary Fig. S1 ) as that by sires isolated with mates ( Fig. 2a ), but without significant changes before and after separation. As the stereotyped retrieval behaviour established over 3 days with pups was abolished by a very brief (10-min) period of separation in a new cage (representing a new environment), as shown in Fig. 1z , the temporal nature of the extinguished parental retrieval behaviour was examined ( Fig. 2b ; n =24 families tested at each time point). When isolated alone for 5–30 min in new cages and then returned to the old cages with five pups, the sires showed little or no pup retrieval behaviour ( Fig. 2b , alone). However, when the sires were housed with their mates in new cages, the retrieval of the five pups in the old cages temporally decreased after 3- and 5-min isolations but recovered after 10- or 30-min isolations ( Fig. 2b , with mate). In sharp contrast, the dams’ retrieval of five pups in the old cages was not significantly decreased by isolation in the new cages with or without sires for any period from 3 min up to 30 min ( Fig. 2c ). Social interaction of paternal males in a three-chambered box To provide an alternative examination of the above effect, the behavioural activity of the parental males was studied in the social interaction chamber shown in Fig. 3 . Experimentally naive sires were removed from their families and placed in the centre room of the apparatus either alone (experiment I, Fig. 3a ) or with their mates (experiment II, Fig. 3c ) for 3, 5 or 10 min. The preference was then examined by tracing their movements for 10 min in the three compartments with five pups in the left chamber ( Fig. 3e ). Sires that had cohabited with their mates for 3, 5 and 10 min showed a relatively constant preference among the three chambers ( Fig. 3h , with mate, n =20, analysis of variance (ANOVA), P <0.05, 0.01 or 0.001, respectively), probably owing to a ceiling or floor effect related to their locomotion when interacting with pups. On the contrary, 20 sires isolated alone gradually exhibited a preference to the left (pups) side and, finally after 10 min, a significant preference for spending time in the empty chamber ( Fig. 3g , alone; ANOVA, P <0.05). 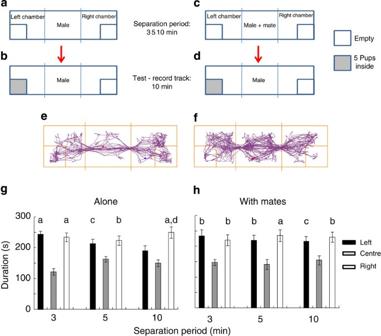Figure 3: Social interaction of parental male ICR mice with pups in a three-chambered apparatus. (a–d) Schematic views of the social interaction chamber. New sires were separated from pups either alone (a, experiment I) or with their mates (c, experiment II) for 3, 5 or 10 min in a central compartment in the Perspex box. Then, five pups were placed in the left compartment (filled box); the opposite compartment was empty (open box), and the sire was then placed alone in the centre compartment. The movements of the sire were recorded online using tracking software. (e,f) Two representative traces of the sires’ movements during social exploration with pups in the left compartment and in the empty cylinder on the right, after separation for 10 min. Left, experiment I (b); and right, experiment II (d). (g,h) By analysing the time spent in three chambers as a function of the isolation period, social preference of the sires was quantified when they were isolated alone (g;n=20), or isolated with their mates (h;n=20). Filled, grey and white bars represent time spent in left, centre and right chambers, respectively (mean±s.e.m.). One-way ANOVA followed by Bonferroni’spost hoctest, the letters (a-c) above the bars indicate significant difference from duration in the central room atP<0.001,P<0.01 andP<0.05, respectively, and (d) denotes significant difference from the left zone atP<0.05. Figure 3: Social interaction of parental male ICR mice with pups in a three-chambered apparatus. ( a – d ) Schematic views of the social interaction chamber. New sires were separated from pups either alone ( a , experiment I) or with their mates ( c , experiment II) for 3, 5 or 10 min in a central compartment in the Perspex box. Then, five pups were placed in the left compartment (filled box); the opposite compartment was empty (open box), and the sire was then placed alone in the centre compartment. The movements of the sire were recorded online using tracking software. ( e , f ) Two representative traces of the sires’ movements during social exploration with pups in the left compartment and in the empty cylinder on the right, after separation for 10 min. Left, experiment I ( b ); and right, experiment II ( d ). ( g , h ) By analysing the time spent in three chambers as a function of the isolation period, social preference of the sires was quantified when they were isolated alone ( g ; n =20), or isolated with their mates ( h ; n =20). Filled, grey and white bars represent time spent in left, centre and right chambers, respectively (mean±s.e.m.). One-way ANOVA followed by Bonferroni’s post hoc test, the letters (a-c) above the bars indicate significant difference from duration in the central room at P <0.001, P <0.01 and P <0.05, respectively, and (d) denotes significant difference from the left zone at P <0.05. Full size image In addition, although it is difficult to correctly monitor sniffing from trace recordings, we estimated the immobilization time in interacting zones ( Supplementary Fig. S2 ). The immobilized time was significantly increased in the left interacting zone with pups, but not in the right zone without pups, by sires isolated with mates for 10 min ( Supplementary Fig. S2B ; n =20, F 2,52 =6.45, P <0.01), while this tendency was not observed in sires isolated alone ( Supplementary Fig. S2A ). These results suggest that cohabitation with maternal mates appears to be important for keeping males’ social approach behaviour to pups, probably by the dam’s signals issued to the sire during the separation period. Therefore, we sought to determine the nature of these putative signals. Cues for paternal care induction In experiments in which the parents were separated into new cages for 10 min ( Fig. 4a–b ), direct contact between the dam and sire was prevented by placing the dam in a transparent plastic box with an open-top ( Fig. 4c ). This arrangement allowed visual, auditory and olfactory cues to pass between the parent mice. Use of this setup did not affect the proportion of sires exhibiting parental care (7 sires retrieved out of 12 subjects tested; 58.3%,) ( Fig. 4d ). When the dams were placed in a transparent plastic box with a lid that blocked transmission of auditory and olfactory stimulation ( Fig. 4f ), paternal care was significantly reduced (1 sire out of 12 families, 8%; Fig. 4g–i ) (Fisher’s test, two-tailed P <0.05). The results of these experiments suggest that paternal behaviour is evoked by exogenous stimuli that occur without direct physical contact, in accordance with a previous study performed in the biparental California mouse [8] . 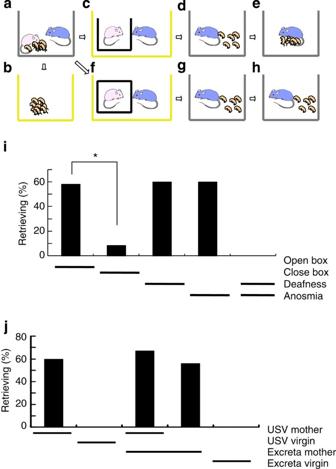Figure 4: Paternal parental behaviour in the separation paradigm under various conditions. (a–h) A schematic representation of the care behaviour test in a mouse pair housed in the same cage (c,f) and isolated from pups in (b) and away from the home nursing cages (a). During the 10-min separation, the parental female was housed either in an open-top box (c) or in a close box (f). The male was then reunited with the pups (d,g), and his subsequent retrieval behaviour (one trial per male) was observed (e,h). (i) Percentage of sires with retrieval responses. The first two columns show responses when the dam was placed in the open-top (c) or sealed box (f). Columns 3–5 show the retrieval behaviour by sires with deafness (with wax ear plugs), anosmia (with 5% ZnSO4solution poured into both nostrils) or both.N=12 sires each, Fisher’s test, two-tailed, *P<0.05. (j) Acoustic and olfactory cues independently induced paternal parental behaviour. USVs were recorded for 10 min from a dam in a new cage with a sire after his removal from a home cage or from virgin females; USVs from the maternal mate (columns 1 and 3) were then played back in a soundproof chamber to the father of the same couple in a new cage (column 1) or in the cage that had previously housed the dam (excreta; column 3). Sires were exposed either to USVs from virgins in a new cage (column 2) or only to the virgins’ excreta (column 5), as above. The sires were then scored for retrieval behaviour when they were returned to their old home cages with pups.N=9–15 subjects, Fisher’s test, two-tailed, *P<0.05. Figure 4: Paternal parental behaviour in the separation paradigm under various conditions. ( a – h ) A schematic representation of the care behaviour test in a mouse pair housed in the same cage ( c , f ) and isolated from pups in ( b ) and away from the home nursing cages ( a ). During the 10-min separation, the parental female was housed either in an open-top box ( c ) or in a close box ( f ). The male was then reunited with the pups ( d , g ), and his subsequent retrieval behaviour (one trial per male) was observed ( e , h ). ( i ) Percentage of sires with retrieval responses. The first two columns show responses when the dam was placed in the open-top ( c ) or sealed box ( f ). Columns 3–5 show the retrieval behaviour by sires with deafness (with wax ear plugs), anosmia (with 5% ZnSO 4 solution poured into both nostrils) or both. N =12 sires each, Fisher’s test, two-tailed, * P <0.05. ( j ) Acoustic and olfactory cues independently induced paternal parental behaviour. USVs were recorded for 10 min from a dam in a new cage with a sire after his removal from a home cage or from virgin females; USVs from the maternal mate (columns 1 and 3) were then played back in a soundproof chamber to the father of the same couple in a new cage (column 1) or in the cage that had previously housed the dam (excreta; column 3). Sires were exposed either to USVs from virgins in a new cage (column 2) or only to the virgins’ excreta (column 5), as above. The sires were then scored for retrieval behaviour when they were returned to their old home cages with pups. N =9–15 subjects, Fisher’s test, two-tailed, * P <0.05. Full size image We next looked for evidence regarding the sensory nature of these stimuli and attempted to determine whether the stimuli are auditory [18] , olfactory [19] or both. USV measurements In the open-box ( Fig. 4c ) and shared-cage ( Fig. 1c ) settings, the male mice could receive auditory stimuli from the females in the form of USVs. We made ultrasound recordings to test whether the female mice emitted USVs to their male partners. As shown in Fig. 5a , which presents a representative set of calls from a dam, USVs consisting of short bursts of a complex, upward, downward, harmonic frequency-modulated tone as previously described [18] , [20] , [21] , [22] , [23] , [24] were detected. The unique USVs emitted by the dams had a fundamental frequency between 30 and 40 kHz, a mean peak frequency of 38.7±0.5 kHz ( n =200 calls in 12 dams) and a mean duration of 121±26 ms ( Fig. 5b ). The average number was 5.1±0.8 calls per min during isolation with mates ( n =12 mice) ( Supplementary Table S1 ). The number of vocalizing dams was 12 out of a total of 13 tested. 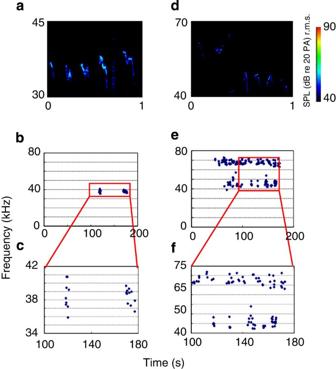Figure 5: USVs emitted by females. USVs emitted by a dam co-housed with a sire during a separation from their pups (a–c) or by a virgin female to another virgin female (d–f). Representative sonograms (a,d) show the acoustic power (sound pressure level, SPL) of the vocalizations as a function of time and frequency (b,cande,f). Note the clusters of very brief USVs of ~38 kHz inbandcand the continuous sounds of two distinct USVs at ~47 and 68 kHz ineandf. r.m.s., root mean squared. Figure 5: USVs emitted by females. USVs emitted by a dam co-housed with a sire during a separation from their pups ( a – c ) or by a virgin female to another virgin female ( d – f ). Representative sonograms ( a , d ) show the acoustic power (sound pressure level, SPL) of the vocalizations as a function of time and frequency ( b , c and e , f ). Note the clusters of very brief USVs of ~38 kHz in b and c and the continuous sounds of two distinct USVs at ~47 and 68 kHz in e and f . r.m.s., root mean squared. Full size image The characteristics of the 38-kHz USVs emitted by the pup-deprived dams were quite different from those of the USVs emitted by virgin female mice of the same age during female–female encounters ( Fig. 5d–f ). Consistent with previous reports [20] , [22] , the latter occurred at a frequency of 81±7 calls per min and consisted of two main components of 47.8±5.2 and 68.4±4.9 kHz ( n =8 mice). The female origin of the USVs was confirmed by anesthetizing the male or female mice as previously reported [22] . USVs were detected when the male mice were anesthetized but not when the females were, indicating that dams emit a series of calls to the sires when deprived of their pups in a new environment. Supplementary Table S1 summarizes that 38-kHz USVs from dams were recorded only under very specific conditions. Thirty-eight kilohertz USVs were not detected when the dam, sire and pups were not manipulated and housed together for 100 min (10 recordings) or when only sires were removed (thus leaving a dam with pups) for 150 min in old cages. Clustered 38-kHz USVs were recorded in one case (out of five) when the sire was reintroduced after 10-min isolation to his old cage with his mate and pups (0.32±0.05 calls per min, Supplementary Fig. S3 ). No 38-kHz USVs were recorded from dams, sires and pups ( n =10) or from dams with pups ( n =5), in which they were transferred into new cages. Thirty-eight kilohertz USVs were not recorded from virgin females that were singly housed continuously in their old cages ( n =5, for 50 min) or in new cages (for 50 min). When a virgin female was exposed to a non-mating sire, USVs of 35–45 KHz were recorded: 1.5±1.3 calls per min ( n =5) in female’s old cages and 2.8±1.8 calls per min ( n =5) in new cages ( Supplementary Fig. S4 ), respectively, though these USVs presumed to be emitted from sires as male’s vocalizations during copulation [18] , [21] . The same 38-kHz USVs were not detected for 100 min from sires alone in old cages when dams and pups had been removed. Induction of paternal behaviour by USV To test whether the 38-kHz USVs emitted by the dams were able to induce parental behaviour in the recipient sires, we first recorded calls emitted for 10 min by the dams during separation from the pups in a new cage with the sires. On the following day, the sires were placed alone in new cages in a soundproof chamber for 10 min and presented with the pre-recorded and unadjusted 10-min calls through a loudspeaker, though the number of USVs varied among the couples. Nine sires retrieved pups out of 15 subjects tested by such replays (60%, Fisher’s test, two-tailed P <0.001 from that with virgin’s USVs; Fig. 4j ). A replay of a 38-kHz sinusoidal (control) noise failed to initiate male parental care ( n =10 sires). Interestingly, as expected, playback of virgin female-to-female USVs did not induce paternal behaviour in the sires (0%, n =10 parental males; Fisher’s test, two-tailed P <0.01). Interaction of auditory and olfactory communication The results of the open-top chamber experiment shown in Fig. 4c suggest that mouse sires may also receive olfactory stimuli from females. To test this hypothesis, we exposed separated sires to the maternal pheromonal stimulation that had been left in cages by dams that had been isolated for 10 min just before the habitation of the sires. This exposure resulted in paternal behaviour in five sires retrieved out of nine (55%, Fig. 4j , Fisher’s test, two-tailed P <0.05 from that with virgin excreta). We then combined the olfactory stimulus with the pre-recorded USVs, which slightly increased male parental behaviour to 67% (8 sires with retrieval out of 12 subjects, Fisher’s test, two-tailed P <0.001 from that with virgin excreta). To further assess the relative effectiveness of auditory and olfactory stimuli in producing parental behaviour, male parents were rendered deaf by the insertion of soft-wax ear plugs or rendered anosmic by intranasal instillation of ZnSO 4 under anaesthesia, as described in Methods. These treatments were effective, as shown in Supplementary Figs S5 and S6 , in separate experiments. Following recovery within 2 h, we tested the effect of these procedures on the male parental response after cohabitation with the female during the separation period, as shown in Fig. 1o ; the results are summarized in Fig. 4i . Deafness and anosmia did not inhibit subsequent male pup retrieval (6 sires with retrieval out of 12 subjects tested in both deafness and anosmia conditions, respectively), but sires subjected to both procedures failed to retrieve their pups (0 sires out of 12; P <0.02, Fisher’s test two-tailed). These results suggest that the USVs and olfactory pheromonal stimuli emitted by females provide essentially equivalent and independent social signals that stimulate neural circuitry [24] , [26] and induce parental behaviour in sires. In this work, we have identified auditory and olfactory signals produced by dams that induce parental behaviour in sires. A 38-kHz USV emitted by dams appears to be a specific signal for stressful conditions, such as separation from pups. The 38-kHz USV is quite distinct from USVs emitted by non-parental females, pups or males ( Fig. 5 , Supplementary Table S1 ; 18, 21, 22) and is sufficient to induce male parental action in the absence of the female ( Fig. 4j ). The 38-kHz USV was supplemented by olfactory signals that may have also contributed to the induction of male parental behaviour during isolation in the home cage. The auditory and olfactory signals were independent and equivalent; together, they were sufficient to induce paternal parental behaviour. We have demonstrated that when male parental mice are continuously housed with their mates and pups for 3–5 days after parturition, the sire exhibits signs of normal female parental care (crouching, licking and pup retrieval). Furthermore, when separated from their pups for 10 min and co-housed with the female parent or kept in the vacated family cage during the separation, male mice showed retrieval behaviour when reunited with the pups. However, male mice housed alone during the separation period did not show retrieval behaviour. The acquisition of retrieval behaviour by co-housed male parents required at least 5–10 min of separation ( Fig. 2b ). Sire behaviour was qualitatively similar to maternal behaviour but was less efficient in that male response levels were slower and less frequent. The 50–60% of sires that showed parental behaviour in this study is similar to the proportion reported in other rodents [2] , [4] , [6] , [7] , [8] , [17] , [27] . Maternal females are enabled to provide ‘focused maternal care’ as a result of co-adaptation of the developing foetus and remodelling of the adult hypothalamus that occurs during parturition [5] , [28] ; this remodelling seems to be irreversible. Recently, Insel [12] proposed that copulation leads to biparental care through activation of vasopressin (V1a) receptors in the ventral pallidum, retrosplenial cortex and anterior hypothalamus, or through the activation of oxytocin and dopamine D2 receptors in the nucleus accumbens (NAcc) in the monogamous pathway. Transient maternal care requires activation of V1a receptors in the lateral septum, oxytocin receptors in the thalamus and dopaminergic receptors in the NAcc in the promiscuous pathway [24] , [26] . The retrieval behaviour of the ICR sires observed in this study was extinguished after a transient 10-min separation in a new environment. This raises the question as to whether inputs from maternal mates to males, rather than copulation, can promote transient care through the signalling pathway suggested. Neural circuits for initiating parental behaviour have been intensively studied in rat dams [29] , [30] . Information from pup stimulation converges on the medial preoptic (mPOA) and ventral tegmental areas as a result of olfactory or oxytocinergic input from the anterior hypothalamic nucleus [31] , [32] . Dopaminergic neurons in the ventral tegmental areas innervate the NAcc [30] . After integration at the NAcc, GABAergic inhibitory signals from the NAcc to the ventral pallidum directly trigger maternal behaviour [24] . Oxytocin receptors are found in the NAcc of spontaneously maternal females [31] . Therefore, it will be interesting to examine which brain areas are important in paternal parental males under this paradigm. A preliminary experiment was performed on quantification of the number of c-Fos immunoreactive cells in male mice with retrieval-positive and retrieval-negative phenotypes to gain a possible neural circuit. When the sires were separated from the pups but kept with a maternal mate, placed in a new cage for 10 min and then euthanized, immunoreactivity was more evident in the mPOA of retrieval-positive sires than retrieval-negative sires. Further experiments are needed to find out if this increased c-Fos expression in mPOA neurons in male parents is likely to be activated by exposure to the maternal mate. In conclusion, in the present work, we have determined the precise conditions associated with paternal parental behaviour in ICR outbred mice. We find an apparently unique susceptibility of sires of the ICR mouse strain to the induction of transient parental behaviour as observed by pup retrieval, and that USVs from dams are one of the factors favouring retrieval responses in sires. The responsiveness shown by sires of the outbred ICR strain should be extended in future studies to other selected mouse lines (inbred and genetically modified) to evaluate whether is a robust dam–sire communicative pattern present in the mouse species. Animals Male and female Slc:ICR outbred mice were obtained from Japan SLC Inc. (Hamamatsu, Japan) via a local distributor (Sankyo Laboratory Service Corporation, Toyama, Japan). The offspring of these mice were born in our laboratory colony, weaned at 21–28 days of age and housed in same-sex groups of 3–5 animals until pairing. The animals were paired and kept in our laboratory under standard conditions (24 °C; 12-h light/dark cycle, lights on at 0800 hours) with food and water ad libitum . The mice were housed together continuously in standard mouse maternity cages. The experiments were performed in accordance with the Guidelines for the Care and Use of Laboratory Animals of Kanazawa University. Behavioural testing Virgin males and females were paired at 45–55 days. A single male and a single female were continuously housed together in a standard mouse maternity cage from the mating period until the delivery of pups until postnatal day 3–5. All family units composed of the new sire and dam, and their first litter were experimentally naïve. In the first experiment ( Fig. 1b–e ), one parent was left in the original cage alone or with his or her mate for 10 min, and the removed sire or dam and all of the pups were placed in holding cages. In the second experiment ( Fig. 1n–q ), the sire and/or dam was placed in a clean cage with new woodchip bedding, but the pups were left in the nest in the original cage. The parents remained in the test environment for 10 min ( Figs 1b–d and 3 , 4 , 5 ) or for 3–30 min, as indicated in Fig. 2b . Five pups were then selected from the litter and placed individually at a site remote from the nest in the original cage. The parents were returned separately to the original home cage with the test pups to assess parental behaviour, as shown schematically in Figs 1 f–i , r–u and . Parental retrieval behaviour (latency to retrieve the first pup, total time required to retrieve five pups and percentage of sires or dams exhibiting retrieval) was examined for 10 min following the reunion. Other parental behaviours defined according to Gubernick and Alberts [8] were also examined; the results of these experiments are shown in Fig. 2a and Supplementary Fig. S1 . Animals in this and subsequent experiments were tested only once. In some of the experiments, the parent was kept individually in a transparent plastic box (60 × 60 × 50 mm 3 ) in the separation cage ( Fig. 4c ). Parental males were rendered deaf or anosmic by 0.3–0.5 ml of soft wax (60 °C melted paraffin wax (Histosec DMSO free, Merck Japan, Tokyo)) was poured or by intranasal infusion of 0.06 ml of 5% ZnSO4 (Wako Chemical Co., Osaka, Japan), for the sensory deprivation condition ( Fig. 4i ). Anosmia was confirmed by the loss of preference for pure water intake over isovaleric acid solution [33] and histologically by ablation of the olfactory epithelium in ten sires examined for behaviour ( Supplementary Fig. S6 ). The effectiveness of the deafening procedures used in these experiments was examined by acoustic startle responses in ten mice with or without ear plugs, as shown in Supplementary Fig. S5 . The deafness was <20% of the control, judging from the normalized ratio to control in Supplementary Fig. S5 . Two experimenters were blinded during the course of the testing and scoring of behaviours to minimize unconscious bias and to ensure objectivity and reproducibility. Tests of sociability The social testing apparatus employed was a rectangular three-chambered box ( Fig. 3a–d ). Each chamber was 60 × 20 × 20 cm 3 . Dividing walls made of plastic with small circular openings (4 cm in diameter) allowed access into each chamber. Each new sire that was separated from his pups for the first time was placed in the middle chamber alone or together with his mate and was allowed to explore for 3, 5 or 10 min. Five pups taken from a family cage were then placed in the left chamber and enclosed in a small round wire cage, which allowed nose contact between the bars. The cage was 6 cm in height, with a bottom measuring 8 × 4.5 cm 2 and bars spaced 0.7 cm apart. When both doors to the side chambers were open, the subject was allowed to explore the entire social test box for a 10-min session. Mobility was monitored with a video camera and then stored on a computer using ANY-maze video tracking software (Stoelting Co., Wood Dale, IL, USA). At the end of the first separation, each parental male was tested in a second 10-min session to quantify social preference for the empty chamber or the chamber containing the pups (in the cohabitation case, the mate was removed during this second test). The amount of time spent in each chamber, the number of entries into each chamber and the number of transitions between chambers of the apparatus were determined during the second 10-min session. Measurement of USVs during social interaction The experiments shown in Figs 4j and 5 were performed in a soundproof chamber. Ultrasonic sounds were detected with a condenser microphone (Type 7016; Aco, Tokyo, Japan) and a preamplifier (Type 4116; Aco) designed for the measurement of sound pressure levels between 20 Hz and 90 kHz. A 20-kHz band-pass filter was used to minimize background noise during recordings; however, most wave files still contained a considerable amount of ‘non-USV’ signal. Extraneous noise was identified and removed from the sonograms as much as possible. When the evaluators found an ultrasound signal that was difficult to interpret, the call was evaluated by at least one additional trained observer, and identification required a consensus by all of the evaluators. Each sonogram was then evaluated with a series of automated parameters. The microphone was placed 50 cm above the cage in a soundproof chamber and connected to an amplifier (model UMA-2; Muromachi Kikai, Tokyo, Japan). Acoustic signals were transmitted to a vocalization analyser system (model MK-1500; Muromachi Kikai) equipped with an analogue-to-digital converter (192 kHz), frequency filters, a digital fast-Fourier-transform analyser and signal input–output terminals. Input signals were visualized using a SpectraLAB (Sound Technology Inc., State College, PA, USA) analyser system on a personal computer ( Fig. 5 ). USVs were also recorded with a microphone (SF-12DC) equipped with an amplifier (model DAF1010; DiaMedical System, Tokyo, Japan). USVs were recorded as wave files and analysed; the number of calls, frequency and wave width were measured using a USV monitor (Muromachi Kikai). Click-like sounds ⩽ 40 ms in duration were filtered out. USVs were analysed by two independent observers, and traces were blinded to them to minimize unconscious bias. In some experiments, to identify sound sources, USVs were measured under cohabitation with either sires or dams anesthetized with pentobarbital sodium (20 mg kg −1 ) for about 1 h. Audible USVs USVs with a sound audible to human ears were monitored using a QL apparatus (model 1; Meiwa System, Yokohama, Japan) designed by I.N., which was connected to a microphone (model 4939-A-011; Brüel & Kjær, Nærum, Denmark). The frequency of mouse USVs was reduced to 1/16 or 1/32 (the audible frequency level to human ears) through a speaker. Replay of USVs To record the waveform and spectrogram of actual USVs from females, a dam was housed with her mate in a cage in a soundproof chamber. The microphone was placed 18 cm from the bottom of the cage and aligned with its centre. The basal microphone noise was ~28 dB. High-pass filter processing was used with a corner frequency of 10 kHz. The sampling frequency rate was 192 kHz. The USV was stored through the UMA-2 USV amplifier. On the following day, the sire was placed in a new cage in the soundproof chamber for 10 min (1–4 calls per min). During this time, USVs recorded from its mate were played back; the sire was then tested for retrieval behaviour in the original home cage with five pups ( Fig. 4j ). For playback, a theta speaker (model PT-R100; Pioneer, Tokyo, Japan) was placed inside the soundproof chamber 50 mm above the floor. Electrical signals corresponding to the reproduced ultrasound through the UMA-2 amplifier were supplied to the device as voltage input via a handmade high-frequency power amplifier system with a high-pass filter. The reproduced USV was monitored by an audible QL apparatus. Statistical analysis Either a one- or two-tailed Student’s t -test or Fisher’s exact test was used for single comparisons between two groups. The remaining data were analysed using one-way ANOVA. Post hoc comparisons were performed only when the main effect was statistically significant. P -values for multiple comparisons were adjusted using Bonferroni’s correction. All of the analyses were conducted using STATA data analysis and statistical software (StataCorp LP, College Station, TX, USA). How to cite this article: Liu, H-X. et al . Displays of paternal mouse pup retrieval following communicative interaction with maternal mates. Nat. Commun . 4:1346 doi: 10.1038/ncomms2336 (2013).